East Siberian Arctic inland waters emit mostly contemporary carbon Inland waters (rivers, lakes and ponds) are important conduits for the emission of terrestrial carbon in Arctic permafrost landscapes. These emissions are driven by turnover of contemporary terrestrial carbon and additional pre-aged (Holocene and late-Pleistocene) carbon released from thawing permafrost soils, but the magnitude of these source contributions to total inland water carbon fluxes remains unknown. Here we present unique simultaneous radiocarbon age measurements of inland water CO 2 , CH 4 and dissolved and particulate organic carbon in northeast Siberia during summer. We show that >80% of total inland water carbon was contemporary in age, but pre-aged carbon contributed >50% at sites strongly affected by permafrost thaw. CO 2 and CH 4 were younger than dissolved and particulate organic carbon, suggesting emissions were primarily fuelled by contemporary carbon decomposition. Our findings reveal that inland water carbon emissions from permafrost landscapes may be more sensitive to changes in contemporary carbon turnover than the release of pre-aged carbon from thawing permafrost. Inland waters are highly abundant and important pathways for the export of terrestrial carbon (C) in northern high-latitude permafrost landscapes where ~50% (~1300 Pg C) of the global soil organic C pool is stored [1] , [2] . This C is increasingly vulnerable to destabilization and release due to permafrost thaw driven by rising Arctic air temperatures [2] , [3] , [4] . Inland waters in stable permafrost landscapes primarily receive terrestrial C from contemporary biological turnover within seasonally thawed topsoils [5] , [6] , [7] . As these landscapes warm, it is likely more contemporary C will be released to inland waters from sustained and enhanced biological turnover and event-based vegetation die-off (Arctic greening versus browning) [8] , [9] . As permafrost soils thaw, additional old C that had remained frozen since the Holocene is also released to inland waters [7] . Twenty-five percent of permafrost soil C is located in regions with substantial deposits of even older, ancient Pleistocene-aged sediments called Yedoma that is particularly vulnerable to thaw due to its high ice content, the majority of which is located in northeast Siberia [1] . These contemporary terrestrial C and old and ancient (pre-aged) C sources are released to inland waters in four main forms: dissolved and particulate organic C (DOC < 0.2–0.7 µm in size <POC), dissolved inorganic C (including CO 2 ), and CH 4 (ref. [2] ). Shifts in the ratio of these C forms from one to another, or increases in total inland water C concentrations, can drive the magnitude of potential climate feedbacks [2] , [10] , [11] . Terrestrial C can be readily decomposed to CO 2 and CH 4 during transport and storage in inland waters and this is thought to be an important driver of permafrost landscape C emissions. Radiocarbon ( 14 C) based studies in Yedoma regions have shown that pre-aged C is highly vulnerable to microbial decomposition to CO 2 when released into streams [12] , [13] , [14] , while studies targeting thermokarst lakes (formed from abrupt thaw processes) detected CH 4 emissions as old as 42,900 years before present (yBP) [15] . In contrast, contemporary C dominated emissions to the atmosphere in non-Yedoma permafrost regions [6] , [7] , [16] , [17] , and ice-core studies suggest it is unlikely that large-scale emissions of pre-aged CH 4 from permafrost regions have occurred in the past ~15,000 years [18] . It therefore remains unclear whether the release of pre-aged permafrost C into inland waters is an important driver of landscape-scale C emissions relative to contemporary C turnover. Here we quantify the contributions of pre-aged and contemporary C in all forms to inland waters of a lowland permafrost landscape. Using an isotope mixing model, we determine the age of C contributions to inland water emissions from simultaneous 14 C and concentration measurements of DOC, POC, and dissolved CO 2 and CH 4 across a selection of inland water sites in the continuous permafrost zone of the northeast Siberian tundra (Fig. 1 ). We focus on dissolved CO 2 and CH 4 rather than ebullition (bubble release) because the dissolved gases provide a more spatiotemporally integrated measure of high-latitude inland water greenhouse gas release [19] . The selected sites cover shallow tundra ponds (<0.5 m deep, 3–240 m 2 in area) with very limited access to pre-aged C (sites P01–12), fluvial systems consisting of an irregularly connected pond and a ~5 m wide stream draining a drained lake basin (sites S01–04), two small lakes (<3 m deep, 0.04 and 0.14 km 2 ) in thaw-depression and drained lake basin dominated tundra (sites L06–12), and a thermokarst lake (up to 7 m depth, 0.51 km 2 ; sites L01–05) that is eroding into a Yedoma ridge (Fig. 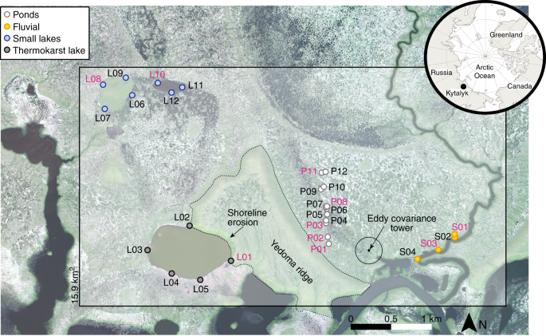Fig. 1: Study region and sampling locations. Sampling locations for concentrations (black text) and radiocarbon (magenta text), eddy covariance tower (black dot) and its footprint (black circle represents 75–90% of flux contributions44), Yedoma ridge (dashed black outline), and location of the site within the Arctic (inset). The box (15.9 km2) indicates the area used for upscaled fluxes (Table1). Background is a panchromatic Worldview satellite image from 15 July 2015, WorldView © 2019 MAXAR. 1 ; Table 1 and Supplementary Table 1 ). 14 C samples were also collected from meltwater draining directly from a thawing Yedoma ice mass in the eroding bank of the thermokarst lake (adjacent to site L01 in Fig. 1 ) to assess the maximum potential age of C mobilized into solution during Yedoma thaw. We expected contemporary C to dominate in the pond, fluvial and small shallow lake sites where inputs of pre-aged C are limited, and pre-aged C to dominate in both the thermokarst lake, which actively erodes into Yedoma sediments, and the Yedoma meltwater. We aimed to capture a snapshot of the likely oldest C released during the growing season by collecting samples in July–August 2016 when the seasonally thawed active layer was deepest and thermokarst erosion was at its maximum (Supplementary Fig. 1 ) [7] , [20] . However, it is worth noting that the oldest C emitted to the atmosphere by such inland waters may occur at the end of winter due to the buildup of CO 2 and CH 4 under ice, which also isolates inland waters from contemporary inputs [19] . Inland water C emissions were upscaled for the 15.9 km 2 study region (Fig. 1 ), and the relative contributions of pre-aged and contemporary C were estimated and contextualized with tundra emissions measured using eddy covariance. The study region is representative of wider northeast Siberian Arctic landscapes, which are dominated by ponds, fluvial networks, drained thaw lake basins and remnant Yedoma deposits [21] , [22] , [23] . Fig. 1: Study region and sampling locations. Sampling locations for concentrations (black text) and radiocarbon (magenta text), eddy covariance tower (black dot) and its footprint (black circle represents 75–90% of flux contributions [44] ), Yedoma ridge (dashed black outline), and location of the site within the Arctic (inset). The box (15.9 km 2 ) indicates the area used for upscaled fluxes (Table 1 ). Background is a panchromatic Worldview satellite image from 15 July 2015, WorldView © 2019 MAXAR. Full size image Table 1 Carbon concentrations/fluxes, upscaled emissions and sources during the study period (25 July–17 August 2016). Full size table Inland water carbon isotope compositions The 14 C ages across the different sampling locations revealed an age gradient ranging from modern (post-1950 CE) to ancient (29,355 ± 2967 yBP; mean ± 1σ; Fig. 2a ): pond sites were the youngest, followed by increasing 14 C ages in the fluvial, small lake, thermokarst lake and Yedoma meltwater sites (Fig. 2b ). Pond, fluvial and small lake 14 C ages were statistically alike, ranging from 1679 ± 38 yBP to modern; thermokarst lake and Yedoma meltwater 14 C ages were significantly older (29,355 ± 2967 to 1234 ± 38 yBP; Fig. 2b ). Fig. 2: Isotope ( 14 C and δ 13 C) composition of all carbon forms. a Dissolved organic carbon (DOC), particulate organic carbon (POC), and dissolved carbon dioxide (CO 2 ) and methane (CH 4 ) across all sample locations; the bars on the left indicate the 14 C (not δ 13 C) values (mean ± 1σ) of the five sources used in the isotope mass balance; 14 C ages are indicative (years before present; yBP); δ 13 C signatures of potential carbon sources are indicated at the top: modern atmospheric CH 4 (ref. [45] ), bacterial methanogensis and bacterial methyl-type fermentation [24] , aquatic (permafrost freshwaters) respiration CO 2 (refs. [19] , [26] ), soil respiration CO 2 and soil organic matter from the study site (including Yedoma soils) [22] , and modern atmospheric CO 2 (ref. [25] ). b 14 C signatures across all carbon forms by sample location; the thick horizontal lines represent the median, limits of the boxes represent upper and lower quartiles, whiskers extend to 1.5 times the interquartile range, dots represent all data points, letters indicate statistical differences between the sample locations using ANOVA (see Methods). Full size image 14 CO 2 values were consistently younger than the other 14 C forms and 14 CH 4 was generally younger than PO 14 C, based on linear regressions testing for age divergence between the different 14 C forms. These regressions were sensitive to extreme values due to limited sample numbers, so thermokarst lake and Yedoma 14 C values were excluded initially. All 14 C forms were significantly correlated with one another ( p < 0.05; R 2 = 0.54–0.94; Supplementary Fig. 2 ). Including the thermokarst and Yedoma samples increased the level of correlation ( p < 0.001; R 2 = 0.74–0.98; Supplementary Fig. 3 ), but CO 2 and CH 4 were still younger than DOC and POC (except thermokarst lake CH 4 and POC, which were approximately the same; Fig. 2a ). The δ 13 C–CO 2 values reflect mixing of respiration of recent and decomposed organic matter with some contribution from methanogenesis as well [24] , [25] . The less negative δ 13 C–CO 2 values (−22.9 to −12.1‰) in comparison with CH 4 were consistent with CO 2 samples collected from Canadian Arctic inland waters [7] . The least negative δ 13 C–CO 2 values indicated there could be some exchange with atmospheric CO 2 which has a less negative δ 13 C value (−9‰) than respired organic matter (−30.0 to −16.2‰) [19] , [22] , [26] , but all sites were supersaturated with CO 2 compared with the atmosphere, limiting ingress of atmospheric CO 2 into the water. The δ 13 C–CH 4 values indicated production from microbial methanogenesis (−63.8 to −46.7‰), although the least negative value was close to thermogenic CH 4 (−45 to −20‰) [24] but this could also reflect enrichment by partial methane oxidation [19] , [24] . The isotopic separation factor ( ε C ) of δ 13 C–CO 2 and δ 13 C–CH 4 (≈δ 13 C–CO 2 − δ 13 C–CH 4 ) can indicate the pathway of CH 4 production. The ε C values in this study were 32.7–45.6 (42.1 ± 4.8 [median ± 1σ]; Supplementary Data 1 ), which indicates CH 4 formation from bacterial methyl-type fermentation (decomposition of methylated organic matter compounds; Fig. 2a ) as opposed to the reduction of carbonate, thermogenic sources, or exchange with the atmosphere [24] . Geological contributions to CO 2 or CH 4 isotopic signatures are very unlikely at the study site (see Methods). The δ 13 C-DOC values (−29.9 to −26.2‰) were consistent with freshwater DOC derived from the C3 photosynthetic pathway [7] , [25] , [27] ; δ 13 C-POC values were more negative (−33.7 to 30.6‰), reflecting the presence of vegetation fragments [25] (Fig. 2a ). Contemporary versus pre-aged carbon sources A five-source isotope mass balance model [6] , [28] , [29] was used to estimate relative contributions to the measured 14 C values from C sources measured at the study site [22] . These C sources were defined as contemporary (modern atmospheric C, topsoil and late-Holocene basal peat: 2013 CE to 1180 yBP) and pre-aged C (old Holocene C and ancient Yedoma C: 1765 yBP to >27,920 yBP) (Fig. 2a ; see Methods). The majority of inland water C observed in this study was contemporary, but pre-aged C contributed to all inland water C forms where permafrost thaw occurred (Fig. 2a ). Pond, fluvial and small lake C was primarily derived from modern and topsoil C sources (>56% ± 33% [mean ± σ]; Fig. 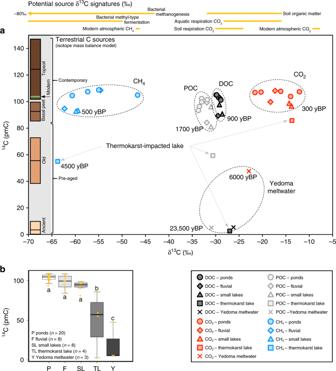Fig. 2: Isotope (14C and δ13C) composition of all carbon forms. aDissolved organic carbon (DOC), particulate organic carbon (POC), and dissolved carbon dioxide (CO2) and methane (CH4) across all sample locations; the bars on the left indicate the14C (not δ13C) values (mean ± 1σ) of the five sources used in the isotope mass balance;14C ages are indicative (years before present; yBP); δ13C signatures of potential carbon sources are indicated at the top: modern atmospheric CH4(ref.45), bacterial methanogensis and bacterial methyl-type fermentation24, aquatic (permafrost freshwaters) respiration CO2(refs.19,26), soil respiration CO2and soil organic matter from the study site (including Yedoma soils)22, and modern atmospheric CO2(ref.25).b14C signatures across all carbon forms by sample location; the thick horizontal lines represent the median, limits of the boxes represent upper and lower quartiles, whiskers extend to 1.5 times the interquartile range, dots represent all data points, letters indicate statistical differences between the sample locations using ANOVA (see Methods). 3 ; Supplementary Table 2 ). When basal peat sources were included, these three contemporary sources accounted for > \(83_{ - 53}^{ + 17}\) % of the C in these waters (Table 1 ). In the thermokarst lake and Yedoma meltwater, the majority of C was pre-aged (>50% ± 35%) (Fig. 3 ; Table 1 ). Fig. 3: Relative source contributions to total inland water carbon. Estimated from a five-source Bayesian isotope mass balance model: modern (2013) atmospheric carbon dioxide (CO 2 ); recent, 1950–2012 carbon fixed into plant and soil organic matter in the topsoil; basal peat ages measured at the site representing the oldest carbon available from Holocene peat accumulation (250–1180 yBP)); old carbon in late-Pleistocene to early Holocene soils (1765–9970 yBP); and ancient Pleistocene-aged Yedoma carbon (>27,920 yBP; Fig. 2a ) [6] , [7] , [22] . Notched lines in the boxes represent the median, limits represent upper and lower quartiles, whiskers extend to 1.5 times the interquartile range, dots represent data points beyond this range. Full size image Carbon concentrations DOC had the highest concentrations of the four C forms measured (15.8 ± 12.3 mg C L −1 [mean ± 1σ]; Fig. 4 ; Supplementary Fig. 4 ). POC and CO 2 concentrations were statistically alike (2.6 ± 3.0 mg C L −1 versus 2.8 ± 3.2 mg C L −1 ), lower than DOC but higher than CH 4 (0.1 ± 0.3 mg C L −1 ). Pond C concentrations were consistently higher than fluvial, small lake or thermokarst lake sites, with the latter three containing statistically alike concentrations (Fig. 4 ). Yedoma meltwater had the highest organic C concentrations (DOC = 42.5 mg C L −1 , POC = 8.5 mg C L −1 ; Table 1 ). Sites with higher CO 2 concentrations had younger 14 CO 2 ages ( p < 0.05, R 2 = 0.71; the best fit was exponential; Fig. 4c ). While this was the only statistically significant relationship, waters with higher overall C concentrations tended to be younger (Fig. 4 ). Fig. 4: Concentrations of all carbon forms. a Dissolved organic carbon (DOC), b particulate organic carbon (POC), c carbon dioxide (CO 2 ), and d methane (CH 4 ) for each sample location; the thick horizontal lines represent the median, limits of the boxes represent upper and lower quartiles, whiskers extend to 1.5 times the interquartile range, dots represent all data points, letters indicate statistical differences between the sample locations using ANOVA (see Methods). Inset: relationship between 14 C content and carbon concentrations (absorbance at 350 nm [a350] for DOC; Supplementary Fig. 4 ) [46] , excluding Yedoma meltwater (see Methods) (*indicates P < 0.05). Full size image Dissolved organic matter characteristics We used absorbance and fluorescence spectroscopy to determine the source and decomposition pathways of inland water dissolved organic matter (DOM) which includes DOC, the C form with the highest concentrations. DOM can be produced by terrestrial and microbial production or decomposed by microbial degradation and photo-oxidation [30] . 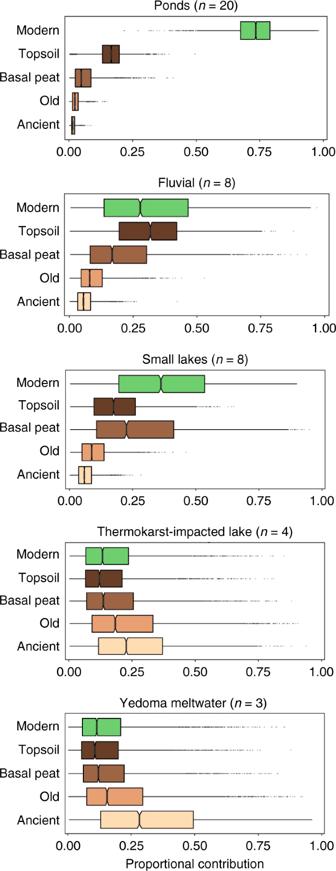Fig. 3: Relative source contributions to total inland water carbon. Estimated from a five-source Bayesian isotope mass balance model: modern (2013) atmospheric carbon dioxide (CO2); recent, 1950–2012 carbon fixed into plant and soil organic matter in the topsoil; basal peat ages measured at the site representing the oldest carbon available from Holocene peat accumulation (250–1180 yBP)); old carbon in late-Pleistocene to early Holocene soils (1765–9970 yBP); and ancient Pleistocene-aged Yedoma carbon (>27,920 yBP; Fig.2a)6,7,22. Notched lines in the boxes represent the median, limits represent upper and lower quartiles, whiskers extend to 1.5 times the interquartile range, dots represent data points beyond this range. 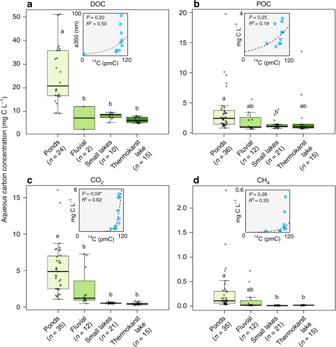Fig. 4: Concentrations of all carbon forms. aDissolved organic carbon (DOC),bparticulate organic carbon (POC),ccarbon dioxide (CO2), anddmethane (CH4) for each sample location; the thick horizontal lines represent the median, limits of the boxes represent upper and lower quartiles, whiskers extend to 1.5 times the interquartile range, dots represent all data points, letters indicate statistical differences between the sample locations using ANOVA (see Methods). Inset: relationship between14C content and carbon concentrations (absorbance at 350 nm [a350] for DOC; Supplementary Fig.4)46, excluding Yedoma meltwater (see Methods) (*indicatesP< 0.05). The DOM was primarily derived from terrestrial material, and both microbial activity and photo-oxidation played a role in its decomposition. Relatively high humic content (Humification Index [HIX] values = 0.6–0.7), indicates a predominantly terrestrial origin, as do substantial contributions of parallel factor analysis (PARAFAC) components C1, C3, and C4 to the total DOM fluorescence signal, which are associated with high aromaticity and intermediate/high-molecular weight terrestrial DOM (Supplementary Fig. 5 ). Higher microbial contributions to the DOM pool were associated with older DOC, indicated by increasing biological index (BIX) values and decreasing humic content with older ages (Supplementary Fig. 6 ). This suggests increased microbial activity that could include the decomposition of organic C to CO 2 and CH 4 , and/or the incorporation of organic C into microbial biomass. Photo-oxidation likely contributed to the decomposition of younger DOM which had higher molecular weight and aromaticity—characteristic of photosensitive molecules [31] —than older DOM. This trend in molecular weight is shown by an increase in S R (slope ratio) and E 2 :E 3 ratio with older ages, both inversely proportional to molecular weight, alongside a decrease in percent C1 (proportional contribution of PARAFAC component C1 to the total fluorescence signal) which is associated with high aromaticity and high-molecular weight terrestrial DOM (Supplementary Fig. 6 ). Landscape-scale carbon emissions The study region was a C sink with a net flux of −876.9 ± 136.4 Mg C during the study period, 25 July–17 August 2016 (summing the upscaled fluxes to the atmosphere in Table 1 ). This was mainly due to the tundra surrounding the inland waters which was a CO 2 sink (−2784 ± 349 mg C–CO 2 m −2 d −1 ) partially offset by tundra CH 4 emissions (43 ± 5 mg C–CH 4 m −2 d −1 ; Table 1 ). 89.4% of the landscape was tundra (14.2 km 2 ; Fig. 1 ), and thus dominated total C flux per unit area and by spatial extent. Of the inland waters, fluvial sites had the highest CO 2 emissions (1820 ± 1118 mg C–CO 2 m −2 d −1 [mean ± 1σ]; Table 1 ; Supplementary Fig. 7 ). Emissions from the pond, small lake and thermokarst lake were all lower than fluvial emissions but not significantly different from one another (290 ± 232 to 394 ± 89 mg C–-CO 2 m −2 d −1 ). The same pattern was evident for CH 4 : fluvial diffusive emissions were 56 ± 29 mg C–CH 4 m −2 d −1 , compared with 18 ± 6 to 20 ± 30 mg C–CH 4 m −2 d −1 from the other sites (Supplementary Fig. 7 ). CO 2 and CH 4 emissions from the fluvial, small lake, and pond fluxes (1.45 km 2 , 7.3% of the study region) were 16.8 ± 10.4 Mg C; the thermokarst lake emissions (0.51 km 2 , 3.2% of the study region) were 3.6 ± 2.8 Mg C. Of these fluxes, contemporary C emissions were 17.0 ± 10.9 Mg C and pre-aged C emissions were 3.5 ± 2.3 Mg C, offsetting 1.9 ± 1.2% and 0.4 ± 0.3% of the tundra sink, respectively. We demonstrate that the inland waters in this permafrost landscape were primarily fueled by contemporary C. We also present direct evidence that pre-aged C can be simultaneously released in all four main inland water C forms where permafrost thaw is occurring. CO 2 and CH 4 tended to be younger than DOC and POC, indicating that contemporary C fuels summer inland water emissions in the study region. This is due to the relatively high abundance of contemporary organic C relative to pre-aged C, and contemporary DOC being more readily photo-oxidized than pre-aged C. The flipside of this finding is that pre-aged inland water C emissions described in previous studies may be caused by the absence of contemporary C as much as by the vulnerability of pre-aged C to microbial decomposition. Given the predominance of labile contemporary C in the inland waters observed in this study, these systems show a high connectivity with contemporary terrestrial C, and are thus likely more sensitive to shifts in contemporary C cycling than the cycling of thawed pre-aged C. Evidence for contemporary C fueling inland waters in this permafrost landscape is demonstrated by the pond, fluvial and small lake sites having the largest upscaled inland water C emissions (equivalent to 2.3 ± 1.5% of the tundra C sink), of which >80% was contemporary C (Table 1 ). In general, sites with higher C concentrations tended to be younger (Fig. 4 ). However, the high proportion of pre-aged C contributing to the thermokarst lake and Yedoma meltwater demonstrates that permafrost thaw will release old and ancient C to all inland water C forms. Across this gradient of inland water 14 C ages (Fig. 2b ), the generally close relationship of CH 4 with DOC and POC with DOC suggests that C release across these different forms was consistently from similar sources. The divergent relationship between DO 14 C/PO 14 C and 14 CO 2 , and PO 14 C and 14 CH 4 was driven by the younger age of the gaseous C (Fig. 2a ). This implies that the C fueling inland water CO 2 and CH 4 emissions was generally younger than mobilized DOC and POC [7] , [32] , and that the most labile organic matter pools were also the youngest. Permafrost thaw can result in high concentrations of low molecular weight DOC and high POC concentrations being released to inland waters [2] , [12] . Incubation-based 14 C studies have suggested that this pre-aged C may be rapidly decomposed to CO 2 (refs. [12] , [13] , [14] ). Our simultaneous in situ 14 CO 2 and 14 CH 4 observations were generally younger than DOC and POC suggesting that contemporary C is also being rapidly decomposed in thaw affected inland waters, potentially at a faster rate or in greater proportion than pre-aged C. The utilization of pre-aged C by microbes previously demonstrated in streams draining thawing ancient Yedoma sediments [12] , [13] , [14] could therefore just be due to the limited availability of contemporary organic C in those systems. This effect is amplified by these studies targeting streams heavily impacted by thermokarst activity, and the incubation approaches used which restrict contemporary inputs entirely. Our findings show that the large amount and high lability of contemporary C mean that it can dominate C cycling compared with thawed pre-aged C in permafrost systems at the landscape-scale. The majority of terrestrial C released into the study inland waters was in the form of DOC (Fig. 4 ) [33] . Our DOM spectroscopy results indicated that the decomposition pathways for DOC was dependent on its source: younger DOC was more vulnerable to photo-oxidation whilst older DOC was more vulnerable to microbial decomposition. Pre-aged permafrost DOC is known to be readily decomposed by microbes [12] , [13] , [14] , and this is supported by the older CO 2 and CH 4 ages observed in our thermokarst lake and Yedoma meltwater (Fig. 2a ). Photo-oxidation can also actively decompose DOC in Arctic inland waters [34] , but is less effective at decomposing ancient Yedoma C [35] . Our samples were collected in late summer when daylight hours can extend for virtually the whole day, so photo-oxidation was likely an important process of organic C decomposition. This is supported by the predominance of contemporary CO 2 and CH 4 , indicating that photo-oxidation of contemporary organic C may be a proportionally more important contributor to inland water emissions in the summer months than microbial decomposition, depending on how much CO 2 and CH 4 is sourced from organic C decomposition in the surrounding soils. Decomposition of pre-aged organic C has most notably been demonstrated in CH 4 ebullition from thermokarst lake sediments that was up to 42,900 yBP in age [15] . In the present study, dissolved CO 2 emissions were larger and younger than dissolved CH 4 , consistent with previously observed Arctic inland water emissions (3–6420 mg C–CO 2 m −2 d −1 versus 1.0–182 mg C–CH 4 m −2 d −1 ) [6] , [7] , [36] , [37] , [38] , [39] , [40] . Both dissolved CO 2 and CH 4 emissions were younger and tended to be smaller than CH 4 ebullition (0–255 mg C–CH 4 m −2 d −1 ) [40] which was not measured in our study. CH 4 ebullition is usually generated at depth, as opposed to dissolved CH 4 which represents a spatiotemporally integrated signal of lake sediment and terrestrial inputs [19] . The generally older age of CH 4 ebullition compared with dissolved CH 4 indicates that where contemporary organic C is limited, such as deep unfrozen lake sediments (taliks), pre-aged C will drive CH 4 production [15] . For example, in Alaskan lakes, dissolved CO 2 and CH 4 collected in winter were older than in summer. This was because frozen lake surfaces prevented inputs of contemporary terrestrial C and stopped ebullition reaching the surface, which allow these bubbles containing old CH 4 and CO 2 to dissolve into the water column (refs. [6] , [19] ). These age differences further indicate that microbial utilization of pre-aged C is due to the restricted supply of contemporary organic C, rather than preferential mineralization of pre-aged organic matter. Inland waters can rapidly turnover contemporary organic C [32] , [41] , and the few existing in situ 14 C measurements of dissolved CO 2 and CH 4 across the Arctic have been contemporary in age [6] , [7] . The export of pre-aged C by inland waters from thawing permafrost landscapes may instead occur as DOC and POC. Our comparison of inland water CO 2 and CH 4 emissions with the measured terrestrial sink does not account for lateral transport of organic C. With DOC and POC concentrations consistently c . 4 times higher and generally older than diffuse CO 2 and CH 4 (Figs. 2 and 4 ), lateral transport is a potentially important component of landscape C loss in the region. Mobilized DOC and POC may be transported laterally to lake, fluvial or marine systems where it can be decomposed to CO 2 and CH 4 , or buried in sedimentary reservoirs [2] , [42] . Rates of lateral transport may be greater at other times of the year than our study period depending on hydrological regimes, e.g., during the Spring snow-melt pulse, and as a result of abrupt thaw events [2] . It is therefore important to track all C forms across different times of the year to fully capture the export of pre-aged permafrost C by inland waters. Our study region had a slightly lower proportional coverage of inland water bodies compared with a selection of Arctic regions in a recent study: of 31 sites, 29 had higher proportional inland water coverage but only by 4.5 ± 3.9% (mean ± 1σ) [23] . Inland waters types and their areal coverage in permafrost landscapes could increase or decrease under climate change depending on localized topography and drainage patterns [4] , [21] , [23] , [43] . There is thus a need to capture C dynamics across a range of water types within the same landscapes, as shown by the variable C concentrations and isotopic compositions seen across our study sites. Our observations demonstrate that inland waters in permafrost landscapes are sensitive to both contemporary and pre-aged C release, although contemporary C dominates in this landscape. This means that regardless of whether the changing Arctic climate will increase inputs of contemporary or pre-aged C to inland waters, their annual CO 2 and CH 4 emissions will likely go up, offsetting terrestrial C sinks. In the study region, inland water CO 2 and CH 4 emissions were a small offset of the terrestrial sink (2.3 ± 1.5% in total), so large increases in inland water coverage and supply of terrestrial C to these waters is needed in order for them to significantly offset the terrestrial sink. Study approach The study site is in the oligotrophic tundra of the Kytalyk Nature Reserve in the Indigirka River lowlands [22] (70.83°N, 147.49°E; Fig. 1 ). Average active layer depths in the tundra around and beneath the ponds during the study period, July–August, were 26 ± 12 cm (mean ± 1σ, n = 370; Table S1 ). The landscape is dominated by a series of drained lake basins formed by thaw driven subsidence and drainage [21] , and the floodplain of the Berelekh River, a major tributary to the Indigirka. A single Yedoma ridge (up to 30-m high) lies within the study region, into which the thermokarst lake is eroding and from which the Yedoma meltwater samples were collected. This ridge is an remnant of organic-rich, ~2–6% C by mass, Pleistocene-aged permafrost sediments deposited as loess or fluvial silts with ice content 30–90% by volume [22] . The ridge covers ~12% of the landscape surface and is potentially distributed throughout the region as a result of thaw and erosion [22] (Fig. 1 ); such deposits are common throughout northeast Siberia [1] . The study region is underlain by continuous permafrost limiting potential geological inputs to aquatic CO 2 or CH 4 , and neither 14 CO 2 nor δ 13 C–CO 2 (which are in isotopic equilibrium with total dissolved inorganic C) correlated with geochemical indicators of rock weathering (e.g., water Ca 2+ concentrations). Geological inputs, such as rock weathering [47] or CH 4 seeps [48] , were therefore unlikely to have influenced our observations. Mean air temperatures during the study period (25 July–17 August 2016) were 10.3 ± 3.3 °C, 7.6 ± 4.7 °C during the growing season (June–September 2016), and −12.4 ± 16.7 °C in the year preceding the sampling campaign. These values are within normal temperature ranges for the site (monthly averages range from 9.7 °C in June to −34.2 °C in January) [22] . Precipitation at the study site occurs mainly as rain during the summer, with an annual mean of 232 mm [22] ; during the sampling period, 30 mm of rain fell compared with 129 mm over the 2016 growing season (Supplementary Fig. 1 ). Vegetation in the tundra areas of the site consists primarily of Eriophorum vaginatum and Eriophorum augustifolium , Betula nana , Carex sp. and Sphagnum sp. The ponds tend to be surrounded by E . vaginatum , E . augustifolium , B . nana , Carex sp., and Sphagnum sp., while the fluvial systems are bordered primarily by Arctophila fulva , Arctagrostis latifolia , and Salix pulchra [49] . Sampling and analyses We collected concurrent 14 C, δ 13 C, and C concentration samples for DOC, POC, and dissolved CO 2 and CH 4 from fluvial, pond, small lake and thermokarst lake sites, and Yedoma meltwater. Samples were collected from the edges of water bodies as could be accessed from the shoreline. Multiple C concentration samples were collected from the lake and stream locations to account for spatial variability. Only one location was sampled for 14 C and δ 13 C in each of the study lakes due to the prohibitive cost of analyses. However, 14 C in dissolved CO 2 and CH 4 have been shown to be relatively uniform in lakes of equivalent size in Alaska [19] . The stream was sampled in two locations and the five different ponds were sampled for 14 C and δ 13 C, but again widespread sampling was limited due to cost. Ponds were only sampled once since their small size means that variations in C source are likely small (Table S1 ). DOC and POC, and dissolved CO 2 and CH 4 concentration samples were collected three times from each site during the study period (except Yedoma meltwater, where n = 1) at three-day intervals in daylight hours for consistency. DOM samples were also collected at the same frequency as the concentration samples but only at sites where 14 C samples were collected (Fig. 1 ; except Yedoma meltwater, where n = 1). 14 C and δ 13 C samples were collected at a single time point from a selection of these sites between 05 and 09 August 2016 (Fig. 1 ; Supplementary Data 1 ) [50] , [51] , [52] , [53] , [54] ; additional δ 13 C samples were also collected for CH 4 and DOC for quality control [55] , [56] , [57] (see Supplementary Methods; Supplementary Fig. 8 ; Supplementary Data 1 and 2 ). Isotope mass balance model The Stable Isotope Mixing Models in R (simmr) package [28] was used to estimate relative contributions of potential C sources to 14 C samples from each group of sample sites (fluvial, pond etc. ; Supplementary Table 2 ). The isotope mass balance model was only used for 14 C because δ 13 C is fractionated during CO 2 and CH 4 production, and so a dual isotope mass balance, common in aquatic organic matter studies [58] , would not work. This approach therefore provides the theoretical possible contributions of different sources following previous studies [6] , [29] , but here the sources are further constrained by using measured soil organic matter 14 C values obtained from the study region [22] . While some water bodies, for example the ponds (see Introduction), are unlikely to receive contributions from pre-aged C sources, we applied the isotope mass balance model with the same end-members to all samples for consistency to demonstrate all possible source contributions that could produce the observed 14 C values. We used simmr to carry out a mass balance (Eq. 1 ), fitting the potential contributions of five different C sources (see below) using Markov chain Monte Carlo modeling. Ranges and uncertainties in the 14 C signature of the different sources were propagated through the model, and model fitting carried out by the Just Another Gibbs Sampler code. Model convergence was only considered acceptable when the upper confidence interval of the final model outputs was 1.00 ± 0.10 (ref. [28] ). We excluded any food web specific functions from the mass balance, such as trophic enrichment factors, or preferential source contributions [28] . C14_group = C14_modern + C14_topsoil + C14_basal peat + C14_old + C14_ancient
 (1) C 14 group represents the 14 C content of the different inland water C components within each group of sample sites (in pmC; Supplementary Data 1 ), which is the sum of the mass balance between the proportional contributions of five different C sources; to achieve mass balance, the relative contributions of the five different sources is assumed to sum to 1. These five sources follow the model used by ref. [6] but is adapted here to incorporate soil/sedimentary 14 C data obtained from the current study site [22] (Fig. 3 ). The modern CO 2 source ( C 14 modern ) was taken as the most recently available atmospheric 14 CO 2 value: calendar year 2013 from Barrow, Alaska (103.13 pmC) [6] , only 3-years earlier than the sampling year in the present study. The topsoil source ( C 14 topsoil ) represents the uppermost soil C accumulation in the peat soils, reflecting atmospheric 14 CO 2 signatures between 1950 and 2012 (123.64 ± 22.61 pmC [mean ± 1σ]) [7] . Basal peat ages ( C 14 basal peat ) represent the oldest C available from the Holocene peat accumulation layers on top of the Yedoma soils (91.95 ± 7.16 pmC) [22] . The old C source ( C 14 old ) represents deep layers of early Holocene to late-Pleistocene C that has come to the surface via cryoturbation (55.13 ± 17.19 pmC) [22] . Ancient C ( C 14 ancient ) represents Pleistocene-aged Yedoma C that has been exposed by thermokarst activity and erosion (3.09 ± 6.19 pmC) [22] . Inland water CO 2 and CH 4 emissions Inland water CO 2 and CH 4 fluxes ( F ) were calculated using Eq. ( 2 ): 
    F = kΔ C
 (2) where Δ C is the difference between the observed gas concentration in the water and the expected concentration if the dissolved gas was in equilibrium with the atmosphere, and k is the gas transfer velocity from water to the atmosphere [59] . Atmospheric CO 2 and CH 4 concentrations were taken from the ambient air samples collected daily during the normal headspace sampling and supplemented with atmospheric concentration data from the eddy covariance tower. Lake k values were calculated using the relationship with wind speed at 10 m ( U 10 in m s −1 ) and k 600 ( k normalized to a Schmidt value of 600) from ref. [60] : 
    k_600 = 2.07 + 0.215 · U_10^1.7
 (3) U 10 values were available from the eddy covariance site at 30 min intervals [49] . Pond k 600 values were taken from ref. [61] (0.36 cm h −1 ), a low k 600 value in the context of inland water k 600 values. Following ref. [59] , for fluvial sites we used the boreal and Arctic stream k 600 value from ref. [62] (13.1 cm h −1 ), which is at the lower end of fluvial k values, but at the high end of inland water k values in general. The k 600 values can then be converted to k : 
    k = k_600/( 600/Sc)^ - 0.5
 (4) where Sc is the Schmidt number in freshwater computed from water temperature [59] . Tundra CO 2 and CH 4 emissions Tundra fluxes at the study site were calculated using the eddy covariance method [63] . The eddy covariance tower at the study site (Fig. 1 ) was installed in 2003 to measure net ecosystem exchange, using an ultrasonic anemometer (Gill Instruments, Lymington, UK, type R3-50) for wind speed and temperature, and water vapor and CO 2 concentrations were measured by an open-path infra-red gas analyzer (LI-COR LI-7500, Lincoln, NE, USA) [49] . An open-path infra-red gas analyzer (LI-COR LI-7700) has been used to measure atmospheric CH 4 concentrations since 2014. All sensors measure at 10 Hz and are installed at a height of 4.7 m. Energy balance closure and good co-spectral shapes required for validation of the eddy covariance methods were demonstrated at the site previously [44] , [49] . Tundra fluxes were calculated via EddyPro (version 6.2.2) to provide 30 min mean fluxes. Processing configuration included: 2D rotation of sonic anemometer coordinates, compensation of air density fluctuations (WPL correction), spectroscopic corrections (for LI7700 – CH 4 flux only) and spectral corrections. Fluxes of CO 2 and CH 4 associated with implausible values of gas concentrations, wind speed or sonic temperature caused by frost, precipitation, water condensation on the analyzer lenses or other conditions of sensors disturbance were removed. CO 2 fluxes were additionally despiked following standard procedure [64] . Daily fluxes (μmol CO 2 m −2 s −1 and nmol CH 4 m −2 s −1 ) were summed and daily standard deviations propagated (by calculating the square root of the sum of squares of daily 1σ uncertainties) for the 23-day study period (25 July–17 August 2016), then converted to a daily C flux (mg C m −2 d −1 ± 1σ; Table 1 ). Values reported in Table 1 are comparable with CO 2 fluxes from the same time period in 2003 to 2013, ranging from −1.4 to −2.3 g C m −2 d −1 , and CH 4 fluxes from the same time period in 2008 to 2015 (pre-2014 fluxes are from chamber measurements at the site) [49] , ranging from 14.5 to 21.0 g C m −2 d −1 . These values are in good agreement with year round fluxes from the site [44] , [49] (Supplementary Fig. 1 ). Upscaling emissions to the study region Daily fluxes measured during the 23-day study period were upscaled to a 15.9-km 2 study area that encompassed all the study sites (Fig. 1 ). The area selected for upscaling captures all the landscape to which we know our measurements apply, i.e., all the lakes, ponds and the stream we sampled plus the surrounding tundra, but we did not try and upscale beyond this. The footprint of the eddy covariance tower captures an area of tundra that reflects the majority of land surrounding the sampled inland water locations, and is considered to be representative of the tundra CO 2 and CH 4 cycling in the immediate region [44] (Fig. 1 ). Areal coverage of the fluvial system (0.2 km 2 ), the small lakes (0.2 km 2 ) and the thermokarst lake (0.5 km 2 ) were calculated from Worldview satellite imagery on 15 July 2015 (Fig. 1 ). Pond coverage was obtained at the study site from satellite imagery and aerial photography from 2002 to 2013 site in a recent study using image classification (4.9 ± 0.2% of the study region) [23] . Daily fluxes of grouped sample locations (fluvial, pond etc.) were multiplied by 23 days and the relative areas of each inland water system to give a total flux to the atmosphere in Mg C for the period 25 July–17 August 2016. 1σ uncertainties in the flux estimates were propagated through the upscaling by providing maximum and minimum values in the total upscaled fluxes ( x ± y in Table 1 ). Relative contributions to fluxes from contemporary (atmospheric, topsoil and basal peat C) versus pre-aged (old and ancient C) sources were estimated by multiplying the fluxes by the proportional contributions of these sources to the total C load (Supplementary Table 2 ). Statistics Statistics were analyzed in R (version 3.5.1). Linear models were used to analyze correlations between groups, and the strength of relationships assessed using analysis of variance (ANOVA), with post hoc Tukey’s honestly significant difference tests (significance level: p < 0.05) carried out using the agricolae package for letters denoting group similarity in, e.g., Fig. 4 . Correlations between variables were assessed using Pearson’s correlations in the Hmisc package (e.g., p -values in Fig. 4 ). Yedoma meltwater values were excluded from the correlation with C concentrations in Fig. 4 (insets) because they represent a Yedoma signal that has yet to be released into an inland water system (unlike the thermokarst lake samples), and because there was no Yedoma 14 CH 4 value, nor CO 2 or CH 4 concentration values, to allow a complete comparison of all correlations.